MicroRNA-302b augments host defense to bacteria by regulating inflammatory responses via feedback to TLR/IRAK4 circuits MicroRNAs (miRNAs) have been implicated in a spectrum of physiological and pathological conditions, including immune responses. miR-302b has been implicated in stem cell differentiation but its role in immunity remains unknown. Here we show that miR-302b is induced by Toll-like receptor 2 (TLR2) and TLR4 through ERK-p38-NF-κB signalling upon Gram-negative bacterium Pseudomonas aeruginosa infection. Suppression of inflammatory responses to bacterial infection is mediated by targeting IRAK4, a protein required for the activation and nuclear translocation of NF-κB. Through negative feedback, enforced expression of miR-302b or IRAK4 siRNA silencing inhibits downstream NF-κB signalling and airway leukocyte infiltration, thereby alleviating lung injury and increasing survival in P. aeruginosa -infected mice. In contrast, miR-302b inhibitors exacerbate inflammatory responses and decrease survival in P. aeruginosa- infected mice and lung cells. These findings reveal that miR-302b is a novel inflammatory regulator of NF-κB activation in respiratory bacterial infections by providing negative feedback to TLRs-mediated immunity. The respiratory system has evolved a potent ability of host defence against bacterial infection. Alveolar epithelial and immune cells, such as macrophages, are the critical components of innate immune system to recognize invading microbes and use inflammatory signals to concert an effective innate and adaptive immune response [1] , [2] , [3] . Gram-negative bacteria are commonly isolated from hospital-acquired infection patients and can cause serious acute and chronic infections in susceptible individuals [4] . The recognition of pathogen-associated molecular patterns by an infected host has been well investigated in recent years [5] , [6] . However, the machinery of innate immune cells that initiates and regulates host immune responses remains incompletely characterized. MicroRNAs (miRNAs) are short regulatory evolutionarily conserved RNAs with the potential to target and suppress multiple genes and linked to most biological functions, such as apoptosis, cell differentiation, cell proliferation and organ development, through diverse signalling pathways comprising biologically meaningful networks [7] . miRNAs can either block mRNA translation or reduce mRNA stability following imperfect binding with the 3′-untranslated regions of target mRNAs [8] . According to the current understanding, individual miRNAs can work via divergent pathways, and the mechanism underlying the repression of protein synthesis by miRNAs is of an intense interest [9] , [10] , [11] . Because the same miRNA can target several transcripts and several miRNAs can also target the same transcript, the miRNA regulatory network appears amazingly complex and challenging. Although miRNAs can constitutively express in different kinds of tissues and changes during development indicate their importance in the maintenance of cellular phenotype, there are also only a small proportion of miRNA targets that have been experimentally validated and the physiological role of the majority of identified miRNAs remains to be fully elucidated [12] , [13] . Recent studies have begun to unravel how miRNAs play key roles in the regulation of diverse biological processes, such as infection, immune response and inflammation. Interestingly, some reports have suggested an important and ancient role for miRNAs in the regulation of the pathogenesis of inflammatory diseases [14] , [15] , [16] . Analyses of individual miRNAs further confirmed important regulatory relationship with specific immune targets in host defence [17] , [18] . Direct roles of miRNAs in innate immune response have been shown in several reports that identified several miRNAs (for example, miR-146a, miR-155 and miR-132) as important regulators in toll-like receptor (TLR) signalling [19] , [20] , [21] , [22] , [23] , [24] . It is our speculation that additional miRNAs may also participate in the immune response and potentially impact the outcome of host–pathogen interaction. Moreover, the detailed mechanisms in regulating host immunity and inflammatory responses by miRNAs are largely unclear. Given the important roles of the TLR signalling pathway in innate antimicrobial immune responses, whether and how TLR signalling and TLR-dependent cytokines production in innate immune cells are regulated by miRNAs warrant deeper investigation. The present study is aimed to investigate whether miRNAs are involved in the regulation of inflammatory responses upon Gram-negative bacterial infection. We use a SYBR Green-based, miScript PCR System to analyse the expression patterns of 84 miRNAs during the activation of alveolar macrophages (AMs), and find that miR-302b is among the most highly induced in the early stage of Gram-negative bacterial infection. Our present data identify that miR-302b, together with other members of miR-302b family, is a crucial regulator of TLRs downstream NF-κB signalling, AMs and epithelial cells activation, and respiratory inflammation by direct targeting IRAK4, a member protein of TLR/MyD88 complex that is critical for NF-κB activation. These results indicate that miR-302b is a novel immunity and inflammatory regulator in respiratory bacterial infection. miR-302b expression is upregulated upon bacterial infection miRNAs have been recently reported as a new regulator in the posttranscriptional regulation of gene expression to play important roles in the regulation of diverse biological processes [25] . To investigate whether the expression of miRNAs might be regulated by P. aeruginosa infection, we analysed the miRNA expression profile of mouse alveolar macrophage MH-S cells (widely used model cells) [3] using an immune response array-based miRNA profiling (catalogue number: MIMM-105, Qiagen, Valencia, CA). After the infection of PAO1 at multiplicity of infection (MOI) 10:1 for 2 h, the array analysis revealed that eight miRNAs were upregulated in macrophages, with miR-302b being the most significantly increased ( Fig. 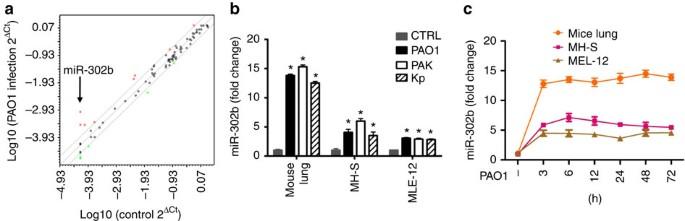Figure 1: miR-302b expression was upregulated after bacterial infection. (a) Microarray analysis of miRNA expression in PAO1-infected MH-S cells versus medium only controls (sham). Genes with >twofold change among subsets andP<0.05 are highlighted (n=3 biological replicates). (b) qRT–PCR analysis of miR-302b expression in lung tissues from the mice, MLE-12 cells and MH-S cells infected with PAO1, PAK and Kp. (c) Time-dependent manner of miR-302b expression in mice lung tissues, MH-S and MLE-12 cells. Mice were treated with 1 × 107CFU of PAO1 and the lung tissues samples (n=5) were collected at different time points from 3–72 h. MH-S and MLE-12 cells were infected with PAO1 at MOI 10:1 for 1 h and polymyxin B (100 μg ml−1) was added for another 1 h to kill bacteria outside of the cells. The cell samples were also collected at different time points from 3–72 h. The miR-302b expression in lung tissues samples, MH-S cells and MLE-12 cells were detected by qRT–PCR. Cell data are representative of three experiments and are shown as means±s.d. (*P<0.05 by one-way analysis of variance with Tukey'spost hoc). Average values and s.d. values for animal data (n=5) were calculated from triplicate samples. 1a and Supplementary Table 1 ). To validate the results of the microarray platform, we determined the expression of miR-302b in MH-S cells infected by two species, three bacteria strains (PAK, PAO1 for P. aeruginosa and Kp for Klebsiella pneumoniae ) by quantitative real time polymerase chain reaction (qRT–PCR). The expression of miR-302b in bacterial-infected cells was determined to be more than threefold higher than that of uninfected cells ( Fig. 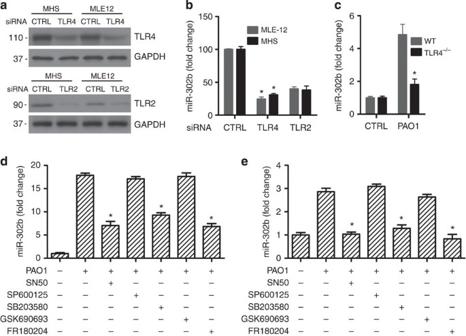Figure 2: miR-302b was induced by TLR2 and TLR4 via the ERK, p38 and NF-κB signalling pathway. (a) MH-S and MLE-12 cells were transfected with control siRNA, TLR4 siRNA or TLR2 siRNA at 10 nM, respectively. Protein lysates prepared at 48 h post transfection were analysed for TLR4 or TLR2 expression by western blotting. (b) 24 h later, the transfected cells were infected with PAO1 at MOI 10:1 for 1 h and polymyxin B (100 μg ml−1) was added for another 1 h to kill bacteria outside of the cells. qRT–PCR analysis of miR-302b expression in MH-S and MLE-12 cells. (c) WT and TLR4−/−mice were infected with 1 × 107CFU per mouse of PAO1 and killed at 12 h post infection (n=3). Lung tissues were lysed to assess the levels of miR-302b. MH-S (d) and MLE-12 cells (e) were cultured for 2 h with medium only (sham) or PAO1 in the presence or absence of SN50, SP600125, SB203580, GSK690693 and FR180204, respectively. The expression of miR-302b was analysed by qRT–PCR analysis. Cell data are representative of three experiments and are shown as means±s.d. (*P<0.05 by one-way analysis of variance with Tukey'spost hoc). Average values and s.d. values for animal data (n=3) were calculated from triplicate samples. 1b and Supplementary Table 2 ). In addition, this result was further confirmed by a robust northern blot analysis ( Supplementary Fig. 1a ). Figure 1: miR-302b expression was upregulated after bacterial infection. ( a ) Microarray analysis of miRNA expression in PAO1-infected MH-S cells versus medium only controls (sham). Genes with >twofold change among subsets and P <0.05 are highlighted ( n =3 biological replicates). ( b ) qRT–PCR analysis of miR-302b expression in lung tissues from the mice, MLE-12 cells and MH-S cells infected with PAO1, PAK and Kp. ( c ) Time-dependent manner of miR-302b expression in mice lung tissues, MH-S and MLE-12 cells. Mice were treated with 1 × 10 7 CFU of PAO1 and the lung tissues samples ( n =5) were collected at different time points from 3–72 h. MH-S and MLE-12 cells were infected with PAO1 at MOI 10:1 for 1 h and polymyxin B (100 μg ml −1 ) was added for another 1 h to kill bacteria outside of the cells. The cell samples were also collected at different time points from 3–72 h. The miR-302b expression in lung tissues samples, MH-S cells and MLE-12 cells were detected by qRT–PCR. Cell data are representative of three experiments and are shown as means±s.d. (* P <0.05 by one-way analysis of variance with Tukey's post hoc ). Average values and s.d. values for animal data ( n =5) were calculated from triplicate samples. Full size image We then investigated whether miR-302b was differentially expressed in bacterial-infected mice versus control mice and bacterial-infected murine lung epithelial cell line MLE-12 versus uninfected control cells ( Fig. 1b ). The results revealed that miR-302b was also upregulated in bacterial-infected mice and MLE-12 cells compared with uninfected counterparts. To validate the expression of miR-302b, we also determined its levels by northern blot analysis that is consistent with the above results, and observed higher expression of miR-302b in bacterial-infected mice ( Supplementary Fig. 1b ) and MLE-12 cells ( Supplementary Fig. 1c ) versus their control mice and cells, respectively. These findings suggest that miR-302b is involved in the infectious process of P. aeruginosa. miR-302b is induced by TLR2 and TLR4 signalling It has been demonstrated that TLR4 and TLR2 play a prominent role in bacterium-induced inflammatory responses [26] . Considering the regulatory mechanism for miR-302b, we hypothesized that TLR4 and TLR2 could induce the expression of miR-302b. MH-S macrophages (phagocytizing bacteria) and MLE-12 epithelial cells (secreting cytokines), which are widely used to study respiratory host defence and immunity in cell culture models [3] , [27] , [28] , [29] were chosen to evaluate their host defence function and were transfected with control siRNA, TLR4 siRNA or TLR2 siRNA at 50 nM, respectively ( Fig. 2a and Supplementary Fig. 2a ). Twenty-four hours after transfection, MH-S and MLE-12 cells were infected with PAO1 and miR-302b expression was detected by qRT–PCR analysis. We found that induction of miR-302b by bacterial challenge was significantly impaired in both TLR4- or TLR2-silenced MH-S and MLE-12 cells ( Fig. 2b ), suggesting that bacteria-induced miR-302b expression was dependent on TLR4 or TLR2. As TLR4 showed more significant changes, we evaluated miR-302b levels in TLR4 knockout mice. Importantly, we observed that bacterial-induced miR-302b expression was impaired in TLR4-deficient mice compared with wild-type (WT) C57BL/6J mice (the same genetic background) ( Fig. 2c ), strongly indicating that TLR4 is involved in miR-302b-mediated immunity against Gram-negative infection. Figure 2: miR-302b was induced by TLR2 and TLR4 via the ERK, p38 and NF-κB signalling pathway. ( a ) MH-S and MLE-12 cells were transfected with control siRNA, TLR4 siRNA or TLR2 siRNA at 10 nM, respectively. Protein lysates prepared at 48 h post transfection were analysed for TLR4 or TLR2 expression by western blotting. ( b ) 24 h later, the transfected cells were infected with PAO1 at MOI 10:1 for 1 h and polymyxin B (100 μg ml −1 ) was added for another 1 h to kill bacteria outside of the cells. qRT–PCR analysis of miR-302b expression in MH-S and MLE-12 cells. ( c ) WT and TLR4 −/− mice were infected with 1 × 10 7 CFU per mouse of PAO1 and killed at 12 h post infection ( n =3). Lung tissues were lysed to assess the levels of miR-302b. MH-S ( d ) and MLE-12 cells ( e ) were cultured for 2 h with medium only (sham) or PAO1 in the presence or absence of SN50, SP600125, SB203580, GSK690693 and FR180204, respectively. The expression of miR-302b was analysed by qRT–PCR analysis. Cell data are representative of three experiments and are shown as means±s.d. (* P <0.05 by one-way analysis of variance with Tukey's post hoc ). Average values and s.d. values for animal data ( n =3) were calculated from triplicate samples. Full size image The stimulation of immune cells by TLR2 and TLR4 ligands can contribute to the activation of the downstream signalling, such as p38, c-Jun NH2-terminal kinase (JNK), ERK, AKT and NF-κB [30] . To identify the pathways that regulate miR-302b expression in MH-S and MLE-12 cells, we pretreated these cells with a set of inflammatory regulator blockers: an NF-κB inhibitor (SN50), an AKT inhibitor (GSK690693), a p38 inhibitor (SB203580), an ERK inhibitor (FR180204) and a JNK inhibitor (SP600125), respectively, and then infected with PAO1 for 2 h. After confirming the inhibition of the targeting gene activity, we measured miRNA expression and showed that inhibition of p38, ERK or NF-κB reduced the induction of miR-302b both in MH-S cells ( Fig. 2d ) and MLE-12 cells ( Fig. 2e ). Therefore, it is likely that miR-302b expression may be regulated by the p38, ERK and NF-κB pathway as a relatively early component of the innate host response. miR-302b represses bacterium-induced inflammatory responses To determine the potential role of miR-302b in bacterial infection, we examined the effect of miR-302b on bacterium-induced inflammatory cytokine gene expression in MLE-12 cells. Using our previously reported methods [31] , we generated useful experimental models to over- or underexpress miR-302b in target cells. Using the chemically synthesized mimics (302b-m)-inhibited bacterium-induced IL-1β, interleukin-6 (IL-6) and tumor necrosis factor alpha (TNF-α) mRNA expression by more than 50% compared with miRNA mimic negative control (NS-m), while miR-302b inhibitors (302b-i) increased these cytokine expressions by ~30% compared with miRNA inhibitor negative control (NS-i) as assessed by qRT–PCR ( Fig. 3a,b , Supplementary Fig. 3 , and Supplementary Table 2 ). In agreement with these results, the protein levels of IL-1β, IL-6 and TNF-α were also lower in cells overexpressing miR-302b than those in cells overexpressing the NS-m as assessed by western blotting. By contrast, the protein levels of IL-1β, IL-6 and TNF-α were higher in the presence of the 302b-i ( Fig. 3c and Supplementary Fig. 2b ). To delve into the detailed mechanisms of innate immune response, we next investigated expression of miR-302b at various time points and demonstrated its time-dependent effect on bacterium-induced inflammatory cytokine gene expression in MLE-12 cells. As shown in Supplementary Fig. 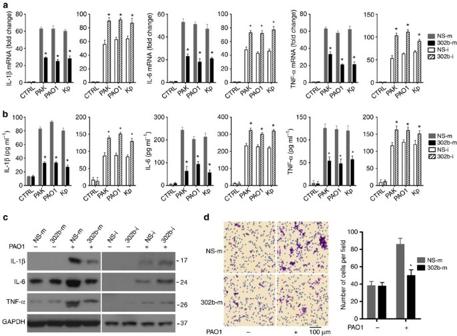Figure 3: miR-302b repressed bacterium-induced proinflammatory cytokine gene expressionin vitro. (a) qRT–PCR analysis of IL-1β, IL-6 and TNF-α mRNA levels in MLE-12 cells transfected with miRNA-negative control (NS-m) or miR-302b mimics (302b-m), miRNA inhibitor negative control (NS-i) or miR-302b inhibitor (302b-i), respectively and infected with PAO1, PAK and Kp. (b) ELISA analysis of IL-1β, IL-6 and TNF-α protein levels in cell culture medium 16 h after PAO1, PAK and Kp treatment. MLE-12 cells were transfected as indicated in (a). (c) Western blot analysis of IL-1β, IL-6 and TNF-α in MLE-12 cells transfected with NS-m or 302b-m, NS-i or 302b-i, after treatment with PAO1, PAK and Kp treatment for 8 h. Densitometry was performed and fold changes of protein expression are shown below the corresponding band. (d) Transwell assay for MH-S cells plated on the upper cell culture inserts, with culture medium from untreated-MLE-12 cells, MLE-12 cells transfected with NS-m or 302b-m as indicated in (b) in the lower chambers. Scale bars, 100 μm. These data are representative of three experiments and are shown as means±s.d. (*P<0.05 by one-way analysis of variance with Tukey'spost hoc). 4 , the peak of the expression of IL-1β was at 6 h; while both of the peaks of the expression of IL-6 and TNF-α were at 2 h. The suppressive function of miR-302b on bacterium-induced inflammatory cytokine gene expression in MLE-12 cells could sustain from 1 to 24 h. Figure 3: miR-302b repressed bacterium-induced proinflammatory cytokine gene expression in vitro . ( a ) qRT–PCR analysis of IL-1β, IL-6 and TNF-α mRNA levels in MLE-12 cells transfected with miRNA-negative control (NS-m) or miR-302b mimics (302b-m), miRNA inhibitor negative control (NS-i) or miR-302b inhibitor (302b-i), respectively and infected with PAO1, PAK and Kp. ( b ) ELISA analysis of IL-1β, IL-6 and TNF-α protein levels in cell culture medium 16 h after PAO1, PAK and Kp treatment. MLE-12 cells were transfected as indicated in ( a ). ( c ) Western blot analysis of IL-1β, IL-6 and TNF-α in MLE-12 cells transfected with NS-m or 302b-m, NS-i or 302b-i, after treatment with PAO1, PAK and Kp treatment for 8 h. Densitometry was performed and fold changes of protein expression are shown below the corresponding band. ( d ) Transwell assay for MH-S cells plated on the upper cell culture inserts, with culture medium from untreated-MLE-12 cells, MLE-12 cells transfected with NS-m or 302b-m as indicated in ( b ) in the lower chambers. Scale bars, 100 μm. These data are representative of three experiments and are shown as means±s.d. (* P <0.05 by one-way analysis of variance with Tukey's post hoc ). Full size image To determine the consequence of miR-302b level changes on the gene expression of inflammatory factors, we detected in vitro migration of macrophages using a Boyden chamber assay. We quantified migration by staining the nuclei of the migratory cells on the underside of insert membrane. As expected, the culture medium from PAO1-infected MLE-12 cells transfected with NS-m markedly increased the migration capabilities of MH-S cells, whereas the medium from miR-302b overexpressed MLE-12 cells decreased the migration of MH-S cells by ~50% ( Fig. 3d ). Moreover, we tested whether miR-302b can regulate the expression of antiinflammatory cytokine genes (for example, Th2). Interestingly, neither the mRNA levels nor the protein levels of IL-4 and IL-10 were significantly altered in MLE-12 cells that overexpressed and underexpressed miR-302b ( Supplementary Fig. 5 ). Taken together, these findings suggest that miR-302b is able to specifically downregulate the expression of proinflammatory genes as well as the migration of macrophages. To dissect the physiological impact of altered miR-302b levels, we further investigated whether systemic administration of miR-302b could inhibit bacterium-induced gene expression in vivo . 302b-m or NS-m was administrated via tail vein of C57BL/6J mice 24 h prior to PAO1 infection. At 12 h after PAO1 infection, the mRNA level of IL-1β was found to be induced by ~12-fold, 9-fold, 4-fold and 5-fold in the lung, liver, heart and spleen tissues in the presence of control mimics. Importantly, administration of miR-302b mimics potently inhibited the induction of IL-1β mRNA expression ( Fig. 4a ). In addition, the expression of IL-6 and TNF-α mRNA also significantly decreased in the lung, liver, heart and spleen ( Supplementary Fig. 6 ). To further verify the observed effects on cytokine mRNA expression, the levels of IL-1β, IL-6 and TNF-α protein in the lung and in bronchoalveolar lavage (BAL) fluid were measured by western blot and enzyme-linked immunosorbent assay (ELISA), respectively. As shown in Fig. 4b and Supplementary Fig. 2c , the protein levels of IL-1β, IL-6 and TNF-α significantly decreased in the 302b-m-treated mice compared with those of control mice. These results were further validated by a standard ELISA ( Fig. 4c ). To determine whether miR-302b contributes to a leukocyte accumulation, histological alteration was also evaluated by hematoxylin and eosin staining. As shown in Fig. 4d,e , miR-302b could reduce leukocyte recruitment in PAO1-infected 302b-m-treated mice compared with that in control mice, consistent with the in vitro data about phagocyte migration and suggesting that macrophage recruitment to the infection site may be influenced by miR-302b. 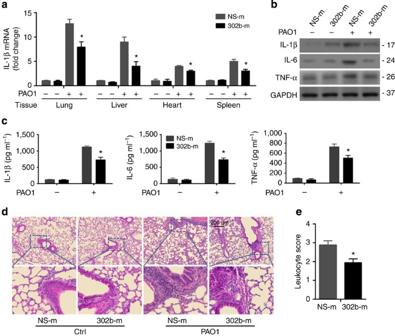Figure 4: miR-302b inhibited bacterium-induced inflammatory responsesin vivo. Mice were i.v. injected with NS-m or 302b-m (50 μg per mouse). Twenty-four hours later, mice were treated with or without 1 × 107CFU of PAO1 for 12 h (a) qRT–PCR analysis of the IL-1β mRNA level in indicated tissues was performed. (b) Lungs were harvested for western blot analysis of IL-1β, IL-6 and TNF-α protein levels. Densitometry was performed and fold changes of protein expression were quantified. (c) BAL fluid was collected and different cytokines were measured by a standard ELISA (eBioscience, Carlsbad, CA). (d) Lung inflammation as assessed by morphologic analysis. The lungs were embedded in formalin and sections were analysed by hematoxylin and eosin staining. Scale bars, 200 μm. (e) Leukocyte infiltration score in lungs. These data are representative of five animals in each group. Error bars indicate±s.d. (*P<0.05 by one-way analysis of variance with Tukey'spost hoc). Figure 4: miR-302b inhibited bacterium-induced inflammatory responses in vivo . Mice were i.v. injected with NS-m or 302b-m (50 μg per mouse). Twenty-four hours later, mice were treated with or without 1 × 10 7 CFU of PAO1 for 12 h ( a ) qRT–PCR analysis of the IL-1β mRNA level in indicated tissues was performed. ( b ) Lungs were harvested for western blot analysis of IL-1β, IL-6 and TNF-α protein levels. Densitometry was performed and fold changes of protein expression were quantified. ( c ) BAL fluid was collected and different cytokines were measured by a standard ELISA (eBioscience, Carlsbad, CA). ( d ) Lung inflammation as assessed by morphologic analysis. The lungs were embedded in formalin and sections were analysed by hematoxylin and eosin staining. Scale bars, 200 μm. ( e ) Leukocyte infiltration score in lungs. These data are representative of five animals in each group. Error bars indicate±s.d. (* P <0.05 by one-way analysis of variance with Tukey's post hoc ). Full size image miR-302b alters the AM cell inflammatory responses to PAO1 AM cells have been reported to play an important role in host defence by phagocytizing bacteria and releasing superoxide [32] . To measure the activity of macrophages, MH-S cells were first transfected with 302b-m, NS-m, 302b-i and NS-i respectively. Next day, the transfected cells were infected with PAO1-GFP at MOI 10:1 for 1 h and the fluorescence intensity was calculated. The results showed that 302b-m or 302b-i-transfected MH-S cells had no changes in phagocytosis ability after infection compared with control reagents-treated cells ( Fig. 5a ). The viability of MH-S cells transfected with 302b-m or 302b-i was also determined by 3-(4,5-dimethylthiazol-2-yl)-2,5-dimethyltetrazolium bromide (MTT) assays. Our data again showed that survival of 302b-m- or 302b-i-transfected MH-S cells was not altered compared with control reagents-treated cells following infection ( Fig. 5b ). However, protein levels of IL-1β, IL-6 and TNF-α in 302b-m transfected MH-S cells significantly decreased when compared with those of NS-m-transfected cells. In contrast, in cells transfected with 302b-i, the protein levels of IL-1β, IL-6 and TNF-α were increased ( Fig. 5c ). To assess the effects of miR-302b on the AM cells in vivo , mice were i.v. (intravenously) injected with 302b-m or NS-m. AM cells were collected from BAL fluid and then infected with PAO1-GFP. Consistent with the results of MH-S cells, neither the phagocytosis nor viability of primary AM cells was changed ( Fig. 5d,e ). Notably, the expression of IL-1β, IL-6 and TNF-α in AM cells was significantly decreased ( Fig. 5f ). These results clearly indicate that miR-302b does not directly impact the phagocytosis ability and viability of AM cells, but may significantly alter the AM cell inflammatory responses (migration and inflammatory cytokine secretion) to bacterial infection. 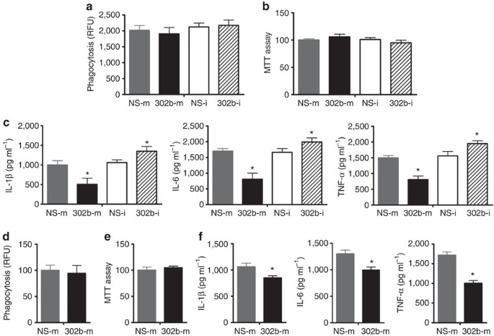Figure 5: miR-302b altered the inflammatory responses of AM cells to PAO1. (a) MH-S cells transfected with NS-m or 302b-m, NS-i or 302b-i. Twenty-four hours later, cells were infected with PAO1-GFP at MOI 10:1 for 1 h. Fluorescence intensity was calculated from triplicate samples. (b) The proliferative ability of AMs from the mice of (a) was measured by the MTT assay. (c) MH-S cells were transfected with NS-m, 302b-m, NS-I or 302b-i for 24 h. Then the cells were infected withP. aeruginosaat an MOI 10:1 for 1 h and polymyxin B (100 μg ml−1) was added for another 7 h. The medium supernatant was collected and different cytokines were measured by a standard ELISA. (d) Mice were i.v. injected with NS-m and 302b-m (50 μg per mouse) for twice. Twenty-four hours after the last dose, AM cells were collected from BAL fluid. The cells were infected with PAO1-GFP at MOI 10:1 for 1 h. Fluorescence intensity was calculated from triplicate samples. (e) The proliferative ability of AMs from the mice of (a) was measured by the MTT assay. (f) AM cells were infected withP. aeruginosaat MOI 10:1 for 1 h and polymyxin B (100 μg ml−1) was added for another 8 h to kill bacteria outside of the cells. The medium supernatant was collected and different cytokines were measured by a standard ELISA. These data are representative of three experiments and are shown as means±s.d. (*P<0.05 by one-way analysis of variance with Tukey'spost hoc). Figure 5: miR-302b altered the inflammatory responses of AM cells to PAO1. ( a ) MH-S cells transfected with NS-m or 302b-m, NS-i or 302b-i. Twenty-four hours later, cells were infected with PAO1-GFP at MOI 10:1 for 1 h. Fluorescence intensity was calculated from triplicate samples. ( b ) The proliferative ability of AMs from the mice of ( a ) was measured by the MTT assay. ( c ) MH-S cells were transfected with NS-m, 302b-m, NS-I or 302b-i for 24 h. Then the cells were infected with P. aeruginosa at an MOI 10:1 for 1 h and polymyxin B (100 μg ml −1 ) was added for another 7 h. The medium supernatant was collected and different cytokines were measured by a standard ELISA. ( d ) Mice were i.v. injected with NS-m and 302b-m (50 μg per mouse) for twice. Twenty-four hours after the last dose, AM cells were collected from BAL fluid. The cells were infected with PAO1-GFP at MOI 10:1 for 1 h. Fluorescence intensity was calculated from triplicate samples. ( e ) The proliferative ability of AMs from the mice of ( a ) was measured by the MTT assay. ( f ) AM cells were infected with P. aeruginosa at MOI 10:1 for 1 h and polymyxin B (100 μg ml −1 ) was added for another 8 h to kill bacteria outside of the cells. The medium supernatant was collected and different cytokines were measured by a standard ELISA. These data are representative of three experiments and are shown as means±s.d. (* P <0.05 by one-way analysis of variance with Tukey's post hoc ). Full size image miR-302b inhibits the activation of NF-κB signalling The expression of proinflammatory cytokine genes is usually mediated by the TLR2 or TLR4 signalling in bacterial infection via the activation of NF-κB, which is a TLR downstream event [26] . To determine whether miR-302b affects NF-κB activation, we next investigated the effect of miR-302b on the phosphorylation of NF-κB p65 subunit in MLE-12 cells. Western blot results showed that the phosphorylation of NF-κB p65 subunit in MLE-12 cells transfected with miR-302b-m was significantly decreased compared with that in the cells transfected with NS-m ( Fig. 6a ). In addition, miR-302b dramatically inhibited the transcription of NF-κB ( Fig. 6b ). As has been well investigated, the translocation of NF-κB from the cytoplasm to the nucleus is an essential step for the transcription of several cytokines [33] . We next explored the effect of miR-302b on NF-κB nuclear translocation using immunofluorescence confocal microscopy. The results showed that NF-κB was activated and translocated into the nucleus in control MLE-12 cells after PAO1 infection but not in miR-302b mimics-transfected MLE-12 cells ( Fig. 6c ). These data suggest that the inhibitory role of miR-302b in bacterium-induced proinflammatory gene expression is due to its effects on the TLR signalling pathway by downregulating the activation of NF-κB. 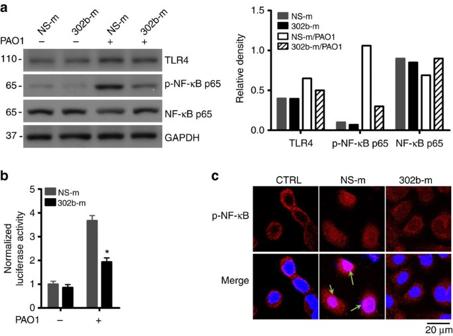Figure 6: miR-302b suppressed the activation of TLR4 signalling pathway. MLE-12 cells were transfected with NS-m or 302b-m for 24 h. Then the cells were infected with PAO1 at MOI 10:1 for 1 h and polymyxin B (100 μg ml−1) was added for another indicated time to kill bacteria outside of the cells. (a) Western blot analysis of TLR4, NF-κB p65 and phosphorylated NF-κB p65 in MLE-12 cells 1 h after PAO1 treatment. Densitometric quantification of the western blotting gel data was used by Quantity one software. (b) Luciferase activity of reporters containing the NF-κB promoter in MLE-12 cells after 12 h infected with PAO1. The cell lysates were subjected to luciferase activity analysis using the Dual-Luciferase Reporter Assay System. (c) Confocal results showed the translocation of p-NF-κB (p-p65) in MLE-12 cells from (a) using immune staining. 4,6-diamidino-2-phenylindole was used to stain the nucleus (arrows showing the nuclear translocation). Scale bars, 20 μm. These data are representative of three experiments and are shown as means±s.d. (*P<0.05 by one-way analysis of variance with Tukey'spost hoc). Figure 6: miR-302b suppressed the activation of TLR4 signalling pathway. MLE-12 cells were transfected with NS-m or 302b-m for 24 h. Then the cells were infected with PAO1 at MOI 10:1 for 1 h and polymyxin B (100 μg ml −1 ) was added for another indicated time to kill bacteria outside of the cells. ( a ) Western blot analysis of TLR4, NF-κB p65 and phosphorylated NF-κB p65 in MLE-12 cells 1 h after PAO1 treatment. Densitometric quantification of the western blotting gel data was used by Quantity one software. ( b ) Luciferase activity of reporters containing the NF-κB promoter in MLE-12 cells after 12 h infected with PAO1. The cell lysates were subjected to luciferase activity analysis using the Dual-Luciferase Reporter Assay System. ( c ) Confocal results showed the translocation of p-NF-κB (p-p65) in MLE-12 cells from ( a ) using immune staining. 4,6-diamidino-2-phenylindole was used to stain the nucleus (arrows showing the nuclear translocation). Scale bars, 20 μm. These data are representative of three experiments and are shown as means±s.d. (* P <0.05 by one-way analysis of variance with Tukey's post hoc ). Full size image IRAK4 is the functional target of miR-302b To identify the molecular target of miR-302b, we searched for predicted miR-302b targets using bioinformatics tools [31] , focusing our attention on the regulators of inflammation. In agreement with this, the public database of the microRNA.org (miRanda) lists IL-1R-associated kinase 4 (IRAK4) as one of the potential targets of miR-302b [34] . IRAK4 has a conservative miR-302b seed sequence in its 3′ UTR ( Fig. 7a ). As a member of IL-1 receptor IRAK family, IRAK4 has been repeatedly demonstrated to be a critical player in TLR-dependent immune responses [35] . These existing knowledge led us to hypothesize that IRAK4 may be a functional downstream target of miR-302b in the inflammatory response to bacterial infection in MLE-12 cells. The expression levels of IRAK4 were first detected in PAO1-infected MLE-12 cells. As shown in Fig. 7b , IRAK4 mRNA expression was reduced by roughly 60% in miR-302b overexpressing cells ( Fig. 7b and Supplementary Tables 2 and 3 ). Additionally, both the total and phosphorylated levels of IRAK4 protein decreased significantly ( Fig. 7c and Supplementary Fig. 7a ). Overexpression of miR-302b inhibited the activity of a luciferase reporter construct containing IRAK4 3′ UTR. In contrast, the activity of luciferase constructs containing the site mutant 3′UTR of IRAK4 was not inhibited by overexpressing miR-302b ( Fig. 7d and Supplementary Table 3 ). To test whether miR-302b post-transcriptionally suppresses the endogenous IRAK4 expression in vivo , we next injected mice with NS-m or 302b-m via i.v. injection. As shown in Fig. 7e,f and Supplementary Fig. 7b , the enforced expression of miR-302b significantly decreased the levels of IRAK4 mRNA, phosphorylated protein and total protein. Thus, our results revealed IRAK4 as a potential target of miR-302b. 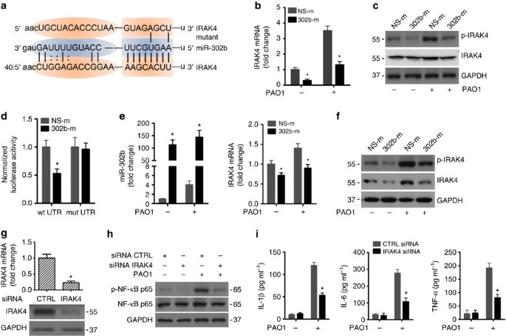Figure 7: IRAK4 is the functional target of miR-302b. (a) IRAK4 3′UTRs contain one predicted miR-302b binding. The figure shows predicted duplex formations between IRAK4 3′UTR (bottom) and miR-302b (middle). The sites of target mutagenesis (top) are also indicated. (b) MLE-12 cells were transfected with NS-m or 302b-m. Twenty-four hours later, cells were infected with PAO1 at MOI 10:1 for 1 h and polymyxin B (100 μg ml−1) was added for another 1 h to kill bacteria outside of the cells. qRT–PCR analysis of IRAK4 mRNA level in MLE-12 cells transfected with NS-m or 302b-m. (c) Western blot analysis of total and phosphorylated IRAK4 protein levels in MLE-12 cells treated as in (b). (d) Normalized luciferase activity of a reporter containing the wild-type or point-mutated 3′ UTR reporter constructs (wt UTR or mutant UTR) of IRAK4 in MH-S cells co-transfected with NS-m or 302b-m. Average values and s.d. values were calculated from triplicate samples. (e,f) Mice were i.v. injected with vehicle, NS-m or 302b-m (50 μg per mouse) for twice times. Twenty-four hours after the last dose, mice were treated with or without 1 × 107CFU per mouse of PAO1 for 12 h. Lungs were harvested for (e) qRT–PCR analysis of the expression of miR-302b and IRAK4 and (f) western blot analysis of total and phosphorylated IRAK4 protein levels. (g) qRT–PCR and western blot analysis of IRAK4 mRNA level in MLE-12 cells transfected with siRNA negative control (NS) or IRAK4 siRNA. (h) Western blot analysis of total and phosphorylated NF-κB p65 in MLE-12 cells treated as in (g). (i) ELISA analysis of elaborated IL-1β, IL-6 and TNF-α protein levels in cell culture medium 16 h after PAO1 infection. MLE-12 cells were transfected as indicated in (g). These data are representative of three experiments and are shown as means±s.d. (*P<0.05 by one-way analysis of variance with Tukey'spost hoc). Figure 7: IRAK4 is the functional target of miR-302b. ( a ) IRAK4 3′UTRs contain one predicted miR-302b binding. The figure shows predicted duplex formations between IRAK4 3′UTR (bottom) and miR-302b (middle). The sites of target mutagenesis (top) are also indicated. ( b ) MLE-12 cells were transfected with NS-m or 302b-m. Twenty-four hours later, cells were infected with PAO1 at MOI 10:1 for 1 h and polymyxin B (100 μg ml −1 ) was added for another 1 h to kill bacteria outside of the cells. qRT–PCR analysis of IRAK4 mRNA level in MLE-12 cells transfected with NS-m or 302b-m. ( c ) Western blot analysis of total and phosphorylated IRAK4 protein levels in MLE-12 cells treated as in ( b ). ( d ) Normalized luciferase activity of a reporter containing the wild-type or point-mutated 3′ UTR reporter constructs (wt UTR or mutant UTR) of IRAK4 in MH-S cells co-transfected with NS-m or 302b-m. Average values and s.d. values were calculated from triplicate samples. ( e , f ) Mice were i.v. injected with vehicle, NS-m or 302b-m (50 μg per mouse) for twice times. Twenty-four hours after the last dose, mice were treated with or without 1 × 10 7 CFU per mouse of PAO1 for 12 h. Lungs were harvested for ( e ) qRT–PCR analysis of the expression of miR-302b and IRAK4 and ( f ) western blot analysis of total and phosphorylated IRAK4 protein levels. ( g ) qRT–PCR and western blot analysis of IRAK4 mRNA level in MLE-12 cells transfected with siRNA negative control (NS) or IRAK4 siRNA. ( h ) Western blot analysis of total and phosphorylated NF-κB p65 in MLE-12 cells treated as in ( g ). ( i ) ELISA analysis of elaborated IL-1β, IL-6 and TNF-α protein levels in cell culture medium 16 h after PAO1 infection. MLE-12 cells were transfected as indicated in ( g ). These data are representative of three experiments and are shown as means±s.d. (* P <0.05 by one-way analysis of variance with Tukey's post hoc ). Full size image To further confirm that IRAK4 is a functional target of miR-302b, we subsequently analysed the effect of IRAK4 on NF-κB activation and the expression of cytokines. As shown in Fig. 7g and Supplementary Fig. 7c , MLE-12 cells transfected with IRAK4 siRNA significantly reduced mRNA levels and protein levels of IRAK4. Importantly, transfection of IRAK4 siRNA into MLE-12 cells resulted in decreased phosphorylation of NF-κB protein compared with that in scrambled siRNA-transfected cells ( Figs 7h-7d ). Moreover, IRAK4 siRNA also reduced the expression of IL-1β, IL-6 and TNF-α compared with that in control siRNA-transfected cells ( Fig. 7i ). Collectively, these data strongly indicate that miR-302b inhibits the NF-κB signalling pathway by directly targeting IRAK4, confirming the functional relevance of this novel target. Decreased IRAK4 mRNA abundance in miR-302b mimic-transfected cells may also be due in part to decreased messenger stability. To address this hypothesis, 24 h after transfection of MH-S and MLE-12 cells with 302b-m and NS-m, we collected cell samples at different time points, extracted their RNA, and detected IRAK4 mRNA abundance by qRT–PCR. As shown in Supplementary Fig. 8 , 302b-m indeed decreased IRAK4 mRNA stability in both MH-S and MLE-12 cells. Lipopolysaccharide (LPS) tolerance is characterized by attenuated macrophage activation and decrease in inflammatory cytokine production during impotent immune defence [36] , [37] . To explore miR-mediated immunity in more detail, we next investigated whether miR-302b affects inflammatory responses to bacterial infection by regulating LPS tolerance in macrophages. Twenty-four hours after transfection of MH-S cells with NS-m, 302b-m, NS-i or 302b-i, the cells were treated with LPS (10 ng ml −1 ) for 24 h and then challenged with 100 ng ml −1 LPS for 2–6 h. The levels of TNF-α (at 2 h) and IL-6 (at 6 h) in culture supernatants were measured by ELISA. The results showed that miR-302b could not regulate the expression of TNF-α and IL-6 in LPS-tolerant MH-S cells ( Supplementary Fig. 9a ). To determine whether miR-mediated immune regulation involves degradation of IRAK, we further detected the ubiquitination of IRAK4 in LPS-treated MH-S cells. We noted that the total ubiquitination and K63 ubiquitination, but not K48 ubiquitination, was decreased in LPS-tolerant MH-S cells ( Supplementary Fig. 9b ). Moreover, we treated NS-m, 302b-m, NS-i and 302b-i-transfected MH-S cells with LPS. There was no significant change of K63 ubiquitination or A20 expression in naive and LPS tolerance in MH-S cells ( Supplementary Fig. 9c ). These data suggest that miR-302b could not regulate LPS tolerance and might not impact ubiquitination to regulate target protein levels. miR-302b decreases susceptibility and mortality rates To determine whether the endogenous expression of miR-302b has any effect on inflammatory responses in vivo , C57BL/6J mice were injected i.v. with 302b-i and then challenged with PAO1. Systemic delivery of miR-302b inhibitors reduced endogenous miR-302b expression by ~70% in lung tissues ( Fig. 8a ). Expression of IL-1β, IL-6 and TNF-α mRNA also increased significantly ( Fig. 8b ). In addition, systemic delivery of 302b-i in mice increased mouse mortality after PAO1 infection over 3 days ( Fig. 8c ). To further dissect the interrelationship between IRAK4 and miR-302b, we also tested the physiological significance in mice models after IRAK4 siRNA and miR-302b mimic treatment. As shown in Fig. 8c , the systemic delivery of IRAK4 siRNA (Ambion In Vivo siRNA) and miR-302b mimic into mice decreased animal mortality from bacterial infection. Moreover, the survival rate of IRAK4 siRNA-treated mice was similarly increased (to a slightly lesser extent) to the mice treated with miR-302b mimics ( Fig. 8c ). Taken together, these results demonstrate a critical role for miR-302b in bacterium-induced inflammatory responses and leukocyte accumulation. Overexpression of miR-302b could represent a novel strategy to negatively regulate the TLR pathways by preventing excessive inflammation that may cause tissue injury or sepsis and may ultimately be beneficial for treating bacterial infection ( Fig. 8d ). 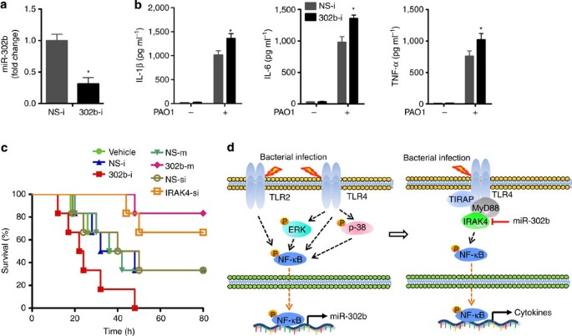Figure 8: miR-302b decreased susceptibility and mortality rate followingP. aeruginosainfection. (a) Mice were i.v. injected with vehicle, NS-i or 302b-i (50 μg per mouse) 24 and 48 h before bacteria challenge. Then, the mice were killed 12 h after 1 × 107CFU of PAO1 infection. Lungs were harvested for qRT–PCR analysis of the expression of miR-302b. (b) BAL fluid of the mice from (a) was collected and different cytokines were measured by a standard ELISA. These data are representative of three experiments and are shown as means±s.d. (*P<0.05 by one-way analysis of variance with Tukey'spost hoc). (c) Kaplan–Meier survival curves of PAO1-infected C57BL/6 mice (1 × 107CFU per mouse). Mice were i.v. injected with vehicle, NS-i, 302b-i, NS-m, 302b-m, NS-si (control siRNA), IRAK4-si (IRAK4 siRNA) (50 μg per mouse) 24 and 48 h before bacterial challenge. Survival was determined up to 80 h. (P=0.013, log-rank test,n=6). (d) Schematic model of the critical role of miR-302b in respiratory bacterial infection pathogenesis. miR-302b is induced by TLR2 and TLR4 through the ERK-p38-NF-κB signalling pathway upon Gram-negative bacterial infection. It functions as a negative feedback regulator in TLR signalling by targeting IRAK4. Figure 8: miR-302b decreased susceptibility and mortality rate following P. aeruginosa infection. ( a ) Mice were i.v. injected with vehicle, NS-i or 302b-i (50 μg per mouse) 24 and 48 h before bacteria challenge. Then, the mice were killed 12 h after 1 × 10 7 CFU of PAO1 infection. Lungs were harvested for qRT–PCR analysis of the expression of miR-302b. ( b ) BAL fluid of the mice from ( a ) was collected and different cytokines were measured by a standard ELISA. These data are representative of three experiments and are shown as means±s.d. (* P <0.05 by one-way analysis of variance with Tukey's post hoc ). ( c ) Kaplan–Meier survival curves of PAO1-infected C57BL/6 mice (1 × 10 7 CFU per mouse). Mice were i.v. injected with vehicle, NS-i, 302b-i, NS-m, 302b-m, NS-si (control siRNA), IRAK4-si (IRAK4 siRNA) (50 μg per mouse) 24 and 48 h before bacterial challenge. Survival was determined up to 80 h. ( P =0.013, log-rank test, n =6). ( d ) Schematic model of the critical role of miR-302b in respiratory bacterial infection pathogenesis. miR-302b is induced by TLR2 and TLR4 through the ERK-p38-NF-κB signalling pathway upon Gram-negative bacterial infection. It functions as a negative feedback regulator in TLR signalling by targeting IRAK4. Full size image Other miRNAs have similar function to miR-302b Accumulating studies have reported that miR-302b belongs to the miR-302 family, which comprises five mature miRNAs: miR-302a, miR-302b, miR-302c, miR-302d and miR-367 (ref. 38 ). They have the same seed sequence and, therefore, may target the mRNA of IRAK4 ( Supplementary Fig. 10 ). As shown in Supplementary Fig. 11a , the expression levels of miR-302a, miR-302b, miR-302c and miR-302d in PAO1, PAK or Kp-infected MLE-12 cells were about 2.2-fold to fourfold higher than those in uninfected MLE-12 cells. Expression of miR-302a, miR-302c, miR-302d and miR-367 was determined by qRT–PCR ( Supplementary Tables 2 and 3 ). Since the level of primary miR-367 was very low (~16 times lower than miR-302b) and there was no significant change after bacterial infection ( Supplementary Fig. 11a ), we did not pursue it further. Overexpression of miR-302s inhibited the activity of a luciferase reporter construct containing IRAK4 3′UTR. In contrast, the activity of luciferase constructs containing the site-directed mutant 3′UTR of IRAK4 was not inhibited by overexpressing miR-302s ( Supplementary Fig. 11b ). Consistent with these results, the mRNA and protein levels of IL-6 were lower in cells overexpressing miR-302s than those in MLE-12 cells overexpressing the miRNA-negative control ( Supplementary Fig. 11c ). Taken together, these results strongly suggest that miR-302 family, sharing the same target IRAK4, is involved in the attenuation of inflammatory cytokines expression during lung bacterial infection in mice and in cell culture models. Several miRNAs, such as miR-132, miR-212, miR-146a and miR-155, have also been reported by several independent laboratories to play an important role in regulating TLR signalling [19] , [21] , [24] , [39] , [40] . To determine the potential role of other miRNAs in our bacterial infection models, we checked our microRNA array list and found miR-155 was also included in the microRNA array with 1.95-fold increase after PAO1 infection ( Supplementary Table 1 ). In comparison with the role of miR-302b, we also examined the effect of miR-155 on bacterium-induced inflammatory cytokine gene expression in MLE-12 cells. Interestingly, forced expression of miR-155 using miR-155 mimics (155-m) could also inhibit bacterium-induced IL-1β, IL-6 and TNF-α mRNA expression compared with NS-m. On the other hand, miR-155 inhibitors (155-i) increased these cytokine expressions compared with NS-i as assessed by qRT–PCR ( Supplementary Fig. 12 ). These results established miR-302b as an important regulator of innate immune response during Gram-negative bacterial infection based on the parallel study with miR-155, a previously recognized immune regulatory miRNA. Eradication of invading bacteria is a critical function of the host immune response. However, some Gram-negative bacteria are able to opportunistically evade the immune system by residing within the host cells in susceptible individuals [41] . The synthesis and accumulation of bacterial products in host cells cause severe damage to the affected tissues [42] . Effective host defence against bacterial invasion requires timely induction of appropriate innate immune responses, which also need to be fine-tuned to avoid excessive tissue injury that may be caused by excessive production of inflammatory cytokines [41] , [43] . To this end, negative regulators are very important to avoid excessive inflammation or uncontrolled immune responses. Recently, some negative regulators in TLR mediated-anti-invading pathogens immune response have been reported [44] , [45] , [46] . Some of these will have a single negative effect (for example, small heterodimer partner (SHP) can act as both a repressor of transactivation of the NF-κB subunit p65 and an inhibitor of polyubiquitination of the adaptor TRAF6 (ref. 45 )), whereas others can be both positive and negative in different cells or physiologic conditions. For instance, transforming growth factor b-activated kinase 1 (TAK1) can function as an essential and positive regulator of innate immune signalling in mouse embryonic fibroblasts, T cells and other cells, which negatively regulates cell development and activation of proinflammatory signalling pathways in neutrophils [47] . These recent findings indicate the existence of complex crosstalk between the positive and negative regulation of the signalling pathways. Although these advances have provided us with an overall understanding of the molecular regulation of innate immunity during infection and inflammation, the detailed mechanisms for some old and new negative regulators need to be further studied. The discovery of small non-coding RNAs, such as miRNAs, has greatly expanded our understanding in the regulation of innate immunity, adaptive immunity and inflammatory responses [48] . Recently, several studies have demonstrated that miRNAs might regulate the inflammatory response initiated by innate immunity [19] , [23] , [40] , [49] . Here, we report a novel negative regulatory network for TLR/NF-κB signalling at the level of miRNAs. Importantly, we found that Gram-negative bacterial infection could induce upregulation of miR-302b expression in AMs and epithelial cells through TLR/NF-κB-dependent pathways. Then, we have proved that miR-302b negatively regulates bacteria-triggered proinflammatory cytokine production, thus indicating a new mechanism to counteract the bacterial evasion of innate immune. Further, we have discovered and validated that mouse IRAK4 is a potential target for miR-302b. Mechanistically, inhibition of miR-302b target, IRAK4, could suppress NF-κB-dependent cytokine production. Therefore, we present a new model that bacterial infection is first sensed by TLR and in turn TLR initiates the production of proinflammatory cytokines against bacterial infection; however, at the same time, bacterial infection can also upregulate the expression of miR-302b which in turn inhibits innate anti-bacterial immune response by blocking TLR signalling and TLR-triggered proinflammatory cytokines production, thus providing a balanced immune response. Previous studies showed that the recognition of TLRs to pathogen-associated molecular patterns can initiate protective immune responses. Studies of TLR signalling have also demonstrated that ligation of TLRs induces the recruitment and activation of IRAK4 (refs 50 , 51 ). Upon binding of a TLR/MyD88 complex, IRAK4 can act as a kinase that functions upstream of and phosphorylates IRAK. Then, the phosphorylated IRAK mediates the recruitment of TRAF6 to the receptor complex [52] . The dissociation from the receptor complex, IRAK–TRAF6 complex interacts with and phosphorylates TAK1. The phosphorylation of TAK1 subsequently leads to the activation of NF-κB and JNK, resulting in transcription of proinflammatory cytokines [53] , [54] . In this study, we found that IRAK4 silencing in MLE-12 cells resulted in significantly decreased phosphorylation of NF-κB and reduced the expression of IL-1β, IL-6 and TNF-α compared with that in control cells. Our results are consistent with a recent report that the TLR-IL-1R-induced NF-κB and JNK activation were abolished in IRAK4-deficient cells and IRAK4 kinase-inactive knock-in mice are resistant to LPS- and CpG-induced shock [35] . The miR-302 family is one of the well-studied miRNAs [55] , [56] , [57] , [58] . miR-302s were vigorously investigated as one of the key factors essential for maintenance of embryonic stem cell renewal and pluripotency [59] . The targets of these miRNAs regulate various cellular processes, including cell cycle, epithelial–mesenchymal transition and vesicular transport [55] . When introduced together with the transcription factors OCT4, SOX2 and KLF4 into human or mouse somatic cells, miR-302s can dramatically enhance dedifferentiation to generate induced pluripotent stem cells [55] . Other studies have reported that miR-302s alone can promote dedifferentiation of cancer cells and human hair follicle cells to an iPSC-like state [59] , [60] . However, this is the first time a member of the miR-302 family has been implicated in a respiratory bacterial infection and the related immune response. These five highly homologous miRNAs members share the same seed sequence. Our bioinformatic studies found that IRAK4 mRNA has an 8-mer seed match in its 3′UTR, which predicts IRAK4 as a target of miR-302. Thus, as a representative of the miR-302 family, miR-302b can significantly suppress both protein and mRNA levels of IRAK4. An array of results in this study also revealed that IRAK4 is a functional target of miR-302s, directly impacting outcome of infection both in cell culture and in mice. Besides, miR-302b and IRAK4 show a significant opposing activity upon bacterial infection in mice as well as in MH-S and MLE-12 cells ( Fig. 1c , Supplementary Fig. 8 ) in a time-dependent manner. However, because a single miRNA may have multiple target genes [61] , whether the miR-302s are able to regulate the expression of other proteins in bacterial infection remains an open question. Several other miRNAs have been implicated to play an important role in inflammatory response [23] , [24] , [39] , [62] . In addition, recent investigations have demonstrated that miR-146a and miR-155 may impact susceptibility to pulmonary infection via targeting TLR signalling [63] , [64] . Moreover, it has been reported that miR-132 and miR-212 could regulate TLR2-mediated tolerance and cross-tolerance through IRAK4 (ref. 24 ). To evaluate whether miR-302b influences LPS tolerance, we used 10 ng ml −1 LPS pretreatment to successfully induce tolerance, but did not observe a significant impact of miR-302b on LPS tolerance ( Supplementary Fig. 9A ). Mechanistically, we examined the role of ubiquitination in our model and found that miR-302 does not require ubiquitin pathways for regulating the IRAK4-mediated innate immunity. Thus, it is logical to propose that a complex circuit may exist in the regulation of innate immunity during Pseudomonal infection. It is tempting to speculate that immune regulatory miR-146a, miR-155 and miR-132 may also be involved in our model. To test this concept, we selected miR-155 as a representative, as this miRNA was included in our array panel with an increase of about twofold after PAO1 infection. Forced expression of miR-155 using miR-155 mimics inhibited bacterium-induced mRNA expression of IL-1β, IL-6 and TNF-α compared with NS-m-transfected controls, while miR-155 inhibitors promoted expression of these cytokines compared with NS-i-transfected controls as assessed by qRT–PCR. Overall, the results strongly indicate that miR-302b is an important regulator of innate immune responses during Gram-negative bacterial infection based on its negative modulation of inflammatory response in vitro and in mice, which is strongly supported by the parallel study with miR-155, a previously recognized immune regulatory miRNA. At this point, we cannot exclude miR-146a and miR-132 as a potential regulator for anti-Pseudomonal immune responses. Thus, this study has added miR-302b and its family members into the growing list of miRs for regulating immunity and inflammation. Finally, these results imply that additional miRNAs may also be involved in the regulation of the inflammation and innate immunity during Gram-negative bacterial infection in the lung and perhaps other organ systems. In summary, we have identified miR-302b as a cytokine-responsive miRNA that regulates the expression of key NF-κB-regulated genes involved in alveolar macrophage and epithelial cell inflammatory responses to bacterial infection both in vitro and in vivo . These findings also revealed an unexpected mechanistic role for this miRNA in targeting downstream NF-κB signalling by directly targeting IRAK4. These studies support an idea that miR-302b may serve as an important negative regulator of inflammatory responses by controlling critical aspects of respiratory system homoeostasis. Thus, these findings provide an insight into the role of miR-302b in the innate immune reaction against Gram-negative bacteria and may indicate a novel therapeutic approach to combat bacterial infection. Mice C57BL/6 female mice (6–8 weeks) were obtained from the Jackson Laboratory (Bar Harbor, ME). TLR4 knocked-out and WT female mice were kindly provided by Dr Jyotika Sharma (University of North Dakota, Grand Forks, ND). Animals were kept in a specific pathogen-free facility of the University of North Dakota. All animal studies were approved by the UND IACUC committee and performed in accordance with the animal care and institutional guidelines (IACUC approval #1204-4). The animal experimental procedures including treatment, care, killing and endpoint choice followed the ARRIVE reporting guidelines. Primary cells and cell lines Primary AMs were obtained from BAL. The mice expired immediately prior to lavage and the thoracic cavity and trachea were dissected. A small incision was made in the trachea via 1-ml syringe with an angiocath (BD Biosciences, San Diego, CA), and recovered to a sterile tube. The mouse lungs were lavaged three times with 1 ml of phosphate-buffered saline (PBS) containing 1% fetal bovine serum. The retained BALF was centrifuged at 600 g for 5 min at 4 °C. The cell pellets were resuspended in RPMI 1640 supplemented with 10% fetal bovine serum (Invitrogen, Carlsbad, CA) and incubated on culture plate for 1 h in 37 °C/5% CO 2 incubator to allow attachment of macrophages. Non-adherent cells were removed by washing with normal saline. Murine MLE-12 lung type II epithelial cells and MH-S AMs were obtained from American Type Culture Collection (Manassas, VA) and cultured following the manufacturer's instructions. Bacteria preparation and infection experiments The P. aeruginosa WT strain, PAO1, was kindly provided by Dr S. Lory (Harvard University, Boston, MA) [65] . PAK and PAO1-GFP were obtained from Dr G. Pier (Harvard University, Boston, MA) [66] . Klebsiella pneumoniae ( K. pneumonia, ATCC43816) was provided from Dr V. Miller (Washington University, St Louis, MO) [67] . Bacteria were grown for about 16 h in LB broth at 37 °C with shaking. The bacteria were pelleted by centrifugation at 5000 g . Various mammalian cells were changed to antibiotic-free medium and infected by bacteria in an MOI of 10:1 bacteria-cell ratio. Mice were anesthetized with 40 mg kg −1 ketamine and then intranasally instilled 1 × 10 7 colony-forming units of PAO1 in 50 μl PBS as described previously [68] . Mice were monitored for symptoms and euthanized when they were moribund. Transfection with siRNA, miRNA mimics and inhibitors TLR2, TLR4 or IRAK4 siRNA were obtained from Invitrogen (Grand Island, NY). miRNA-negative control (NS-m, Cat #CN-001000-01-05), miR-302a mimics (302a-m, Cat #C-310483-05-0005), miR-302b mimics (302b-m, Cat #C-310669-05-0010), miR-302c mimics (302c-m, Cat #C-310671-05-0005), miR-302d mimics (302d-m, Cat #C-310672-05-0005), miR-155 mimics (155-m, Cat #C-310430-07-0005), miRNA inhibitor negative control (NS-i, Cat #IN-001005-01-05), miR-302b inhibitor (302b-i, Cat #IH-310669-06-0010) and miR-155 inhibitor (155-i, Cat #: IH-310430-08-0005) were obtained from Dharmacon (Chicago, IL). MH-S or MLE-12 cells were transfected with miRNA or siRNA using Lipofectamine 2000 reagent (Invitrogen, Grand Island, NY) for 24 h following the manufacturer's instruction. Mice were i.v. administered with vehicle (in vivo-jetPEI, Polyplus-transfection, New York, NY), IRAK4 siRNA, NS-m, 302b-m, NS-i or 302b-i (50 μg per mouse) twice (24 h and 48 h) before bacteria challenge following the manufacturer's instruction. Measurement of miRNA and mRNA expression Total RNA was extracted using the TRIzol (Invitrogen, Grand Island, NY) according to the manufacturer’s instructions. RNA was eluted in RNase-free water and stored at −70 °C. For non-radioactive northern blot, LNA and DIG-modified miR-302b probe was purchased from Exiqon (Vedbaek, Denmark). The DIG-modified sno202 probes were synthesized by Integrated DNA Technologies (Coralville, IA). The northern blot protocol was performed according to a published protocol as previously described [69] . Real-time PCR profiling of miRNAs were conducted on a SYBR Green-based, miScript PCR System (Cat #MIMM-105, Qiagen, Valencia, CA). The expression of mRNAs was detected by QuantiTect SYBR Green RT–PCR Kit (Qiagen, Valencia, CA). The separate well 2−ΔΔ C t cycle threshold method was used to determine relative quantitative levels of individual miRNAs or mRNA, and these were expressed as the fold difference to the sno202 or GAPDH, respectively. Western blot analysis Mouse monoclonal Abs against GAPDH and IL-6 and goat polyclonal Abs against IL-1β and TNF-α were obtained from Santa Cruz Biotechnology (Santa Cruz, CA). Rabbit monoclonal Ab against phosphor-NF-κB p65, phospho-IRAK4, A20/TNFAIP3, ubiquitin, K48-linked polyUb chains, K63-linked polyUb chains and IRAK4 were purchased from Cell Signaling Technology (Cambridge, MA). The samples derived from cells and lung homogenates were lysed in RIPA buffer, separated by electrophoresis on 12% SDS–PAGE gels and transferred to nitrocellulose (GE Amersham Biosciences, Piscataway, NJ). Proteins were detected by western blotting using primary Abs at a concentration of 1/200 (Santa Cruz Biotechnology) or 1/1,000 (Cell Signaling Technology) and were incubated overnight. Labelling of the first Abs was detected using relevant secondary Abs conjugated to HRP (Santa Cruz Biotechnology, Santa Cruz, CA) and detected using ECL reagents. Histological analysis Lung tissues were fixed in 4% formalin for 24 h and then processed to hematoxylin and eosin staining in AML Laboratories (Baltimore, MD). The numbers of leukocytes were counted using the normal optical microscope. MTT assay Mice were killed at the indicated times after P. aeruginosa infection and the AMs were collected from BAL fluid. Primary AMs or MH-S cells were cultured in a 96-well plate. MTT assay was performed as described previously [68] . In brief, the cells were incubated with MTT (1 μg ml −1 ) after incubation with PAO1 at 37 °C for 4 h. 100 Stop solution (10% SDS in 50 mM HEPES buffer) 100 μl per well was added and the plate was left at 37 °C overnight for complete dissolution of formazan crystals. The plate was read at 570-nm absorbance using a plate reader in the next day. Duplicates were done for each sample and control. Background correction was done with blanks containing dye alone. In vitro migration assay MLE-12 cells were transfected with NS-m or 302b-m for 24 h and infected by PAO1 in a MOI of 10:1 bacteria-cell ratio for 16 h. The culture medium was collected and was placed in the lower chamber. MH-S cells were loaded into the Boyden chamber with an 8 μm porous membrane (Corning) in 100 μl RPMI 1640 medium/1% serum and incubated at 37 °C for 4 h. Cells were removed from the upper side of membranes, and nuclei of migratory cells on the lower side of the membrane were stained with crystal violet. MH-S cells that attached to the filter were counted by light microscopy. Confocal microscopy MLE-12 cells were transfected with miRNA-negative control or miR-302b mimics for 24 h. Cells were infected by PAO1 in a MOI of 10:1 bacteria-cell ratio for 1 h, incubated with primary anti-p-NF-κB p65 Abs, and the second antibodies as described in our previous report. 4′,6-diamidino-2-phenylindole (Sigma-Aldrich, St Louis, MO) was used to stain the nucleus. Luciferase assay Transient transfections were performed with 2 × 10 5 MLE-12 cells plated in 6-well plates by using pNF-κB-luc plasmid (Promega, Madison, WI) following the manufacturer's instruction. Twenty-four hours after transfection, the cells were infected with PAO1 for 12 h. Cell lysates were subjected to luciferase activity analysis by using the Luciferase Reporter Assay System (Promega). Actinomyocin D Treatment of Cells Twenty-four hours after the transfection of the MH-S and MLE-12 cells with 302b-m and NS-m., 5 μM actinomycin D (Sigma-Aldrich, St Louis, MO) was added into the plates. Cells were subsequently harvested at different time points (0, 15, 30, 60, 180, 360 and 720 min). IRAK4 mRNA levels were detected by qRT–PCR. LPS tolerance Twenty-four hours after transfection of MH-S cells with NS-m, 302b-m, NS-i and 302b-i, the cells were pretreated for another 24 h with 10 ng ml −1 LPS, washed with PBS and returned to fresh medium for 2 h. Naive and LPS-pretreated cells were stimulated with 100 ng ml −1 LPS for different time points. IL-6 and TNF-α production was determined by ELISA. IRAK4 was immunoprecipitated from cell lysates, followed by immunoblot analyses with Abs specific for Ubiquitin, K63-linked Ub and for K48-linked Ub chains. Statistical analysis All statistical analyses were done with SPSS 19.0 software. Data are presented as mean±s.d. Statistical analysis was performed by Student’s t -test for comparing two groups and by one-way analysis of variance with Tukey's post hoc for multiple group comparisons. Differences in the mean values were considered to be significant at P <0.05. How to cite this article : Zhou, X. et al. MicroRNA-302b augments host defence to bacteria by regulating inflammatory responses via feedback to TLR/IRAK4 circuits. Nat. Commun. 5:3619 doi: 10.1038/ncomms4619 (2014).